Structure of GrlR–GrlA complex that prevents GrlA activation of virulence genes The locus of enterocyte effacement ( LEE ) is essential for virulence of enterohaemorrhagic Escherichia coli (EHEC) and enteropathogenic E. coli (EPEC). The 41 genes of the LEE encode type III secretion system proteins and three associated regulators: Ler, GrlA and GrlR. Ler is a positive regulator for most of the LEE operons, including grlRA . GrlA controls the expression of ler , ehxCABD and flhDC operons. GrlR binds to GrlA and suppresses its function. Here we report the crystal structure of GrlR–GrlAΔ (aa 1–106) complex (2:1) and its functional characterization. We show that GrlR interacts with the Helix-Turn-Helix motif of GrlA. Moreover, GrlA binds to the promoter DNA fragments of ler , ehxCABD and flhDC , and GrlR outcompetes with these promoter DNA sequences for the Helix-Turn-Helix motif of GrlA. These findings provide mechanistic insight into a regulatory module for the virulence of EPEC and EHEC, two important pathogens that cause devastating diseases. Attaching and effacing (AE) pathogens comprise a group of enteric pathogens, including the closely related enterohaemorrhagic Escherichia coli (EHEC) and enteropathogenic E. coli (EPEC). EPEC causes severe diarrhea in young children, whereas EHEC is a causative agent of haemorrhagic colitis and haemolytic uremic syndrome [1] , [2] . AE pathogens possess type III secretion systems (T3SS) that promote virulence. Most T3SS components and related proteins are encoded by genes in the locus of enterocyte effacement (LEE) . The LEE consists of 41 genes, clustered in 5 different operons, termed LEE1–LEE5 , and some additional transcription units [3] . Under specific conditions, such as low temperature, the histone-like nucleoid-structuring (H-NS) protein binds to extended regions within the LEE DNA and silences the expression of the entire LEE region. This H-NS-mediated repression, however, can be countered by Ler ( LEE -encoded regulator), a protein encoded by the first gene in the LEE1 operon that functions as a positive regulator of other LEE operons ( LEE2–LEE5 ) [4] . Moreover, Ler is involved in both the direct and indirect regulation of additional key virulence components of EPEC and EHEC, and is thus considered as the master regulator of the virulence machineries of these pathogens. Accordingly, activation of LEE1 and ler expression is a key event in the activation of the entire virulence system of EPEC and EHEC. It is therefore not surprising that the LEE1 promoter is subjected to tight regulation by multiple factors ( Fig. 1 ), including H-NS and Ler, which function as repressor and autorepressor, respectively. The expression of the LEE1 operon is strictly dependent on binding of the integration host factor protein immediately upstream to the LEE1 promoter [4] , and activation of LEE1 expression is promoted by two redundant positive regulators, PerC [5] (or Pch in EHEC) and GrlA. 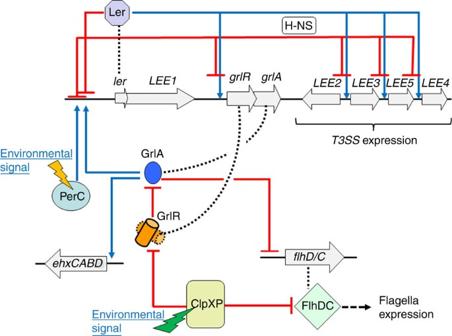Figure 1: Schematic of the regulatory circuits related to the GrlR–GrlA complex. We propose the following model based on results presented in this report as well as results previously published by others and by us. ThegrlRandgrlAgenes form a bicistronic operon located within theLEE. Under non-inducing conditions, the expression of the entireLEE, includinggrlRA, is suppressed by a H-NS protein, and the activity of the residual GrlA is suppressed by GrlR via direct interaction (repression is indicated by red lines). The expression of the entire system can be activated by two alternative modes. The first involves specific environmental cues that turn on PerC expression; this, in turn, activates the expression ofler(activation is indicated by blue lines). Ler then antagonizes H-NS and stimulates the expression of all of the otherLEEoperon components, includinggrlRA. The produced GrlA directly activateslerexpression to establish the GrlA-Ler-positive feedback loop. Consequently, GrlA indirectly promotes the expression of allLEEgenes, directly activates the expression of theehxoperon, and represses the expression of the flagella master regulatorflhDC.The GrlA-Ler loop is restrained by the autorepressive action of Ler as well as by GrlR, which directly binds to GrlA to inhibit its interaction with target DNA. The second mode of activation involves environmental signals that trigger the ClpXP protease to degrade GrlR, thus releasing GrlA to activatelerexpression and mediate the establishment of the Ler-GrlA-positive loop described above. Figure 1: Schematic of the regulatory circuits related to the GrlR–GrlA complex. We propose the following model based on results presented in this report as well as results previously published by others and by us. The grlR and grlA genes form a bicistronic operon located within the LEE . Under non-inducing conditions, the expression of the entire LEE , including grlRA , is suppressed by a H-NS protein, and the activity of the residual GrlA is suppressed by GrlR via direct interaction (repression is indicated by red lines). The expression of the entire system can be activated by two alternative modes. The first involves specific environmental cues that turn on PerC expression; this, in turn, activates the expression of ler (activation is indicated by blue lines). Ler then antagonizes H-NS and stimulates the expression of all of the other LEE operon components, including grlRA . The produced GrlA directly activates ler expression to establish the GrlA-Ler-positive feedback loop. Consequently, GrlA indirectly promotes the expression of all LEE genes, directly activates the expression of the ehx operon, and represses the expression of the flagella master regulator flhDC. The GrlA-Ler loop is restrained by the autorepressive action of Ler as well as by GrlR, which directly binds to GrlA to inhibit its interaction with target DNA. The second mode of activation involves environmental signals that trigger the ClpXP protease to degrade GrlR, thus releasing GrlA to activate ler expression and mediate the establishment of the Ler-GrlA-positive loop described above. Full size image The grlR and grlA genes form a transcriptional unit encoding GrlR and GrlA, respectively. GrlA is a positive regulator of the LEE1 promoter and forms a positive regulatory loop with Ler. GrlR binds to GrlA and this is thought to account for the negative effect of GrlR on ler expression [3] , [4] , [6] . As GrlA and GrlR are co-expressed, it is expected that, in most cases, GrlA is inhibited by GrlR and that the relative levels of GrlR and GrlA are regulated. For instance, it was reported that under certain conditions GrlR is degraded by the ClpXP protease, freeing GrlA to activate Ler expression [7] . Previously, we reported the structure of GrlR and elucidated its role in LEE regulation [8] , [9] . GrlR forms a stable and tight dimer in solution as well as in the crystal. The dimeric architecture of GrlR is maintained by the cluster of hydrophobic interactions as well as numerous hydrogen-bonding contacts at the dimeric interface [8] . GrlA has also been functionally characterized [3] , [4] , [10] , but no structural information is available to provide insight into the regulatory mechanisms involving GrlA, GrlR and Ler. In addition to its function as a LEE1 regulator, GrlA negatively regulates the transcription of the flhDC operon and thus controls flagellar gene expression. Kitagawa et al. [11] demonstrated that flagellar gene expression in EHEC was strictly regulated by dual pathways: (i) post-translational control of the FlhD/C master regulator by ClpXP-mediated protein degradation and (ii) transcriptional control of the flhDC operon through the GrlR–GrlA system under LEE-inducing conditions. Moreover, deletion of grlR results in a non-motile phenotype in the EHEC O157 Sakai strain [6] . In many pathogens, motility is repressed by negatively regulating flhDC concomitant with T3SS induction [11] . GrlA-dependent repression of flagellar regulation is important for efficient adhesion of EHEC to host cells [6] , [11] and perhaps also to avoid detection by the host innate immune sensors TLR5 and NLRP4 (refs 12 , 13 ). GrlA is also implicated in the transcriptional activation of the ehxCABD operon in EHEC [14] , [15] . The ehxA gene encodes haemolysin, and ehxC acts as a modifying factor that converts inactive haemolysin into its active form by the addition of a fatty acid group [16] ; the specific secretion machinery for EhxA is encoded by ehxB and ehxD [17] . The in vitro instability of GrlA has previously hindered structural studies and other attempts to elucidate the regulatory mechanism involving Ler, GrlA and GrlR. Here we report the crystal structure of GrlAΔ (aa1–106) in complex with GrlR, refined up to 2.7 Å resolution, and the associated functional studies. The structure is asymmetric with a stoichiometry of 2 GrlR:1GrlAΔ. In addition, we identify a novel regulatory mechanism by which GrlR interacts with GrlA at its Helix-Turn-Helix (HTH) motif, preventing GrlA from binding to its target promoter DNA. Overall structure of the GrlR–GrlAΔ complex We initially attempted to determine the structure of full-length GrlA in complex with GrlR. However, the full-length GrlR–GrlA complex did not yield diffraction quality crystals, presumably because of the unstable nature of GrlA. As a result, we generated GrlR–GrlA complexes with varying lengths of GrlA. A complex of GrlR with GrlAΔ (aa1–106) ( Fig. 2a ) yielded diffraction quality crystals. The structure was determined and refined up to 2.7 Å resolution ( Table 1 and Fig. 2b ). The first 8 residues and last 11 residues of GrlAΔ were not well-defined in the electron density map and were not included in the model. GrlR is a β-barrel protein, structurally similar to our previously determined GrlR structures (root mean squared deviation (r.m.s.d.) of 0.87 Å for all C α atoms) [8] , [9] , whereas GrlAΔ mainly comprises a HTH motif (aa 39–66) and an anti-parallel β-sheet in the carboxy terminus ( Fig. 2c,d ). The complex consists of one dimer of GrlR bound to a monomer of GrlAΔ (2:1 stoichiometric ratio), with 15 hydrogen-bonding contacts (<3.2 Å) formed between GrlR and GrlAΔ, and a buried area of 1,043.8 Å (ref. 2 ). This GrlR:GrlA stoichiometric ratio was further verified by analytical ultracentrifugation, which showed that the complex is of 47.3 kDa, corresponding to two molecules of 6His-GrlR and one molecule of GrlA ( Fig. 2e ). This is consistent with the gel filtration experiment ( Supplementary Fig. S1a,b ). 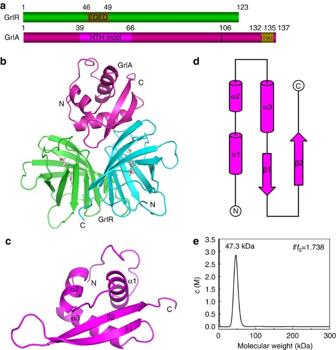Figure 2: Structure of the GrlR–GrlAΔ heterotrimeric complex. (a) GrlR and GrlA proteins with motifs. (b) Crystal structure of the GrlR–GrlAΔ complex. The two monomers of GrlR are shown in green (monomer A) and cyan (monomer B). GrlAΔ is shown in magenta. The ligand Triton X-100 is shown as sticks. (c) Structure of GrlAΔ. (d) The topology diagram of the GrlAΔ molecule. Structure-related figures are prepared using PyMol35. (e) The stoichiometric ratio of WT GrlR–GrlA complex protein was investigated in an analytical ultracentrifuge by monitoring their sedimentation properties in a sedimentation velocity experiment. The peak corresponds to a molecular weight of 47.3 kDa, indicating the presence of two molecules of 6His-GrlR and one molecule of GrlA in the complex. Figure 2: Structure of the GrlR–GrlAΔ heterotrimeric complex. ( a ) GrlR and GrlA proteins with motifs. ( b ) Crystal structure of the GrlR–GrlAΔ complex. The two monomers of GrlR are shown in green (monomer A) and cyan (monomer B). GrlAΔ is shown in magenta. The ligand Triton X-100 is shown as sticks. ( c ) Structure of GrlAΔ. ( d ) The topology diagram of the GrlAΔ molecule. Structure-related figures are prepared using PyMol [35] . ( e ) The stoichiometric ratio of WT GrlR–GrlA complex protein was investigated in an analytical ultracentrifuge by monitoring their sedimentation properties in a sedimentation velocity experiment. The peak corresponds to a molecular weight of 47.3 kDa, indicating the presence of two molecules of 6His-GrlR and one molecule of GrlA in the complex. Full size image Table 1 Crystallographic statistics and refinement details. Full size table Sequence and structural homology of GrlA GrlA homologues are present in over 100 species of bacteria, including EPEC, EHEC, Citrobacter rodentium , Shigella sp. and Salmonella sp. with no structures available to date. GrlA shares 33% sequence identity (46% similarity) with CaiF, a potential transcriptional activator of carnitine metabolism in E. coli , and belongs to the PFAM family of DUF1401 ( http://pfam.sanger.ac.uk/family/DUF1401 ). Despite a very low sequence identity (<7%), the DALI [18] search for structural homologues of GrlA identified several regulatory proteins. The closest homologues are also HTH motif-containing proteins, such as a transcriptional regulator from Methanosarcina mazei (PDB 3R0A; r.m.s.d. 2.8 Å for 72 C α atoms), a DNA-binding protein from Pyrococcus horikoshii OT3 (PDB 1ULY; r.m.s.d. 2.5 Å for 67 C α atoms) and a double-stranded RNA-specific adenosine deaminase (PDB 3F23; r.m.s.d. 2.6 Å for 61 C α atoms). These structural similarities suggest that these homologues may have similar functions, such as in transcriptional regulation. GrlR interacts with the HTH and C-terminal regions of GrlA The crystal structure of the complex revealed that GrlR interacts with the HTH motif region of GrlAΔ ( Fig. 3a,b and Supplementary Fig. S2a,b ). The residues R53, R54, R64, R65 and K66 from the HTH region of GrlAΔ are involved in hydrogen-bonding contacts with GrlR. Our previous studies with GrlA [8] suggested that the C-terminal region of GrlA might be involved in binding to GrlR (please refer to the Discussion section). Therefore, we sought to independently verify the contribution of the amino-terminal HTH motif and the C terminus of GrlA in its interaction with GrlR. To verify this, we created three constructs by substituting the abovementioned five interacting amino acids of the HTH motif region with alanine (denoted as GrlA5M), truncating the C-terminal region of GrlA (GrlAΔ), or both mutations (GrlAΔ5M). Thus, the various GrlA constructs used in these interaction studies include MBP-GrlA, MBP-GrlA5M, MBP-GrlAΔ and MBP-GrlAΔ5M. The circular dichroism spectrum of the wild type (WT) and mutants of GrlA suggest that the mutants have the same fold as the WT GrlA ( Supplementary Fig. S3 ). 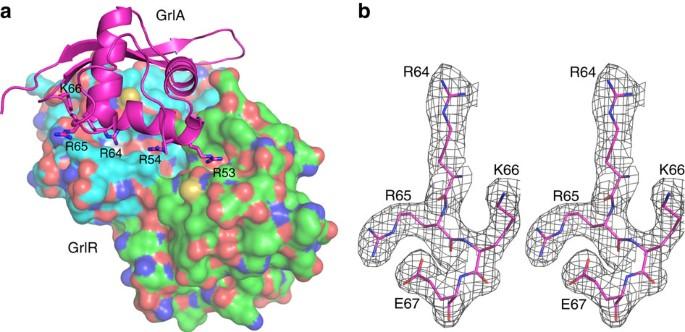Figure 3: Structure of the GrlR–GrlAΔ interacting surface. (a) The GrlR dimer is shown in surface representation and GrlAΔ is shown as a cartoon. The interacting residues of GrlAΔ are shown as sticks. (b) Final2Fo-Fcelectron density map (contoured at 1σ) for the key residues of GrlAΔ. Figure 3: Structure of the GrlR–GrlAΔ interacting surface. ( a ) The GrlR dimer is shown in surface representation and GrlAΔ is shown as a cartoon. The interacting residues of GrlAΔ are shown as sticks. ( b ) Final 2Fo-Fc electron density map (contoured at 1 σ ) for the key residues of GrlAΔ. Full size image The K d for the interaction between GrlR and MBP-GrlA was determined by isothermal titration calorimetry (ITC). GrlR interacts with MBP-GrlA with an ~35-fold higher affinity ( K d =0.031 μM) than with MBP-GrlAΔ ( K d =1.1 μM) ( Fig. 4a and Supplementary Table S1 ). Similarly, the K d for the interaction between GrlR and MBP-GrlA5M was also higher ( K d =0.96 μM) than the WT interaction ( Fig. 4b and Supplementary Table S1 ). Besides the 35- and 31-fold reductions in affinity, respectively, MBP-GrlAΔ and MBP-GrlA5M also showed thermodynamic profiles distinct from the WT MBP-GrlA. Although the MBP-GrlA interaction with GrlR is enthalpically and entropically favourable (Δ H =−4.8 kcal mol −1 and − T Δ S =−5.4 kcal mol −1 ), the other two protein variants (GrlAΔ and GrlA5M) showed an enthalpically driven interaction, with unfavourable entropic contributions (Δ H =−21.0 kcal mol −1 and − T Δ S =12.9 kcal mol −1 , for MBP-GrlAΔ; Δ H =−9.6 kcal mol −1 and TΔS=1.3 kcal mol −1 , for GrlA5M; Supplementary Table S1 ). 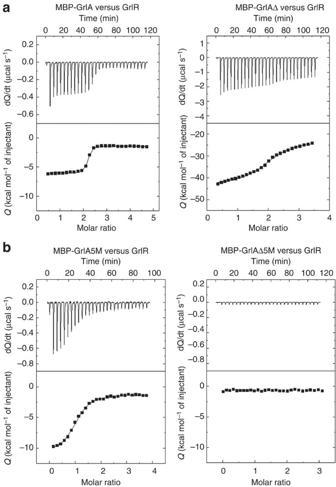Figure 4: Role of the C-terminal region and the HTH motif region of GrlA in GrlR–GrlA interactions. (a) The binding affinities of MBP-GrlA/MBP-GrlAΔ to GrlR were determined using ITC. Representative ITC profiles are shown. The GrlA proteins used are indicated above each panel. The upper part of each panel shows the thermogram (thermal power versus time) after baseline correction and the bottom part of each panel shows the binding isotherm (normalized heat versus molar ratio of reactants) for each injection. The solid lines in the bottom part of each panel show the fit of the data to a function based on a single class of binding site model. (b) The binding affinities of GrlR to MBP-GrlA/MBP-GrlAΔ with substitutions in the HTH motif region (5 M) were determined using ITC (5 M refers to substitutions at R53A, R54A, R64A, R65A and K66A). The binding constants (KaandKd), number of binding sites (N), enthalpy (ΔH) and entropy (ΔS) are provided inSupplementary Table S1. Figure 4: Role of the C-terminal region and the HTH motif region of GrlA in GrlR–GrlA interactions. ( a ) The binding affinities of MBP-GrlA/MBP-GrlAΔ to GrlR were determined using ITC. Representative ITC profiles are shown. The GrlA proteins used are indicated above each panel. The upper part of each panel shows the thermogram (thermal power versus time) after baseline correction and the bottom part of each panel shows the binding isotherm (normalized heat versus molar ratio of reactants) for each injection. The solid lines in the bottom part of each panel show the fit of the data to a function based on a single class of binding site model. ( b ) The binding affinities of GrlR to MBP-GrlA/MBP-GrlAΔ with substitutions in the HTH motif region (5 M) were determined using ITC (5 M refers to substitutions at R53A, R54A, R64A, R65A and K66A). The binding constants ( K a and K d ), number of binding sites ( N ), enthalpy (Δ H ) and entropy (Δ S ) are provided in Supplementary Table S1 . Full size image GrlR interacted with the WT MBP-GrlA or MBP-GrlAΔ with a stoichiometric ratio of 2:1. However, the stoichiometric ratio between GrlR and MBP-GrlA5M was 1:1, which suggests that two MBP-GrlA5M molecules bind with a dimeric GrlR ( Supplementary Table S1 ). The MBP-GrlAΔ5M construct did not show binding to GrlR. Subsequently, we examined the role of each of the aforementioned key residues in mediating the interaction between GrlR and GrlA by pull-down assay. MBP-GrlAΔ containing double amino acid substitutions (MBP-GrlAΔ (R53A R54A), MBP-GrlAΔ (R64A R65A) and MBP-GrlAΔ (R65A K66A)) did not interact with GrlR ( Fig. 5a and Supplementary Figs S4a,b and S5a ), whereas single alanine substitutions had little effect on the GrlAΔ–GrlR interaction ( Supplementary Fig. S5b ). Consistent with the ITC results, MBP-GrlA, MBP-GrlAΔ and MBP-GrlA5M pulled down GrlR, whereas MBP-GrlAΔ5M did not ( Supplementary Fig. S5c ). We further verified the role of the key residues of GrlR in mediating GrlA binding, which shows that alanine substitution at D35 and E60 of GrlR could abolish its binding to MBP-GrlAΔ ( Fig. 5b and Supplementary Fig. S5d ). Moreover, these results were confirmed using a pETDuet-1- grlR-grlA Δ co-expression and co-purification system with 6His tag on GrlR and a tagless GrlAΔ ( Supplementary Figs S6a,b, S7 and S8 ). Taken together, these results show that GrlR–GrlA interaction involves both the HTH motif region and the C-terminal region of GrlA. 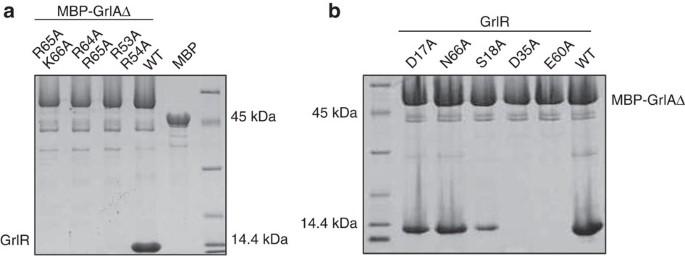Figure 5: Role of the key residues in the HTH motif region in GrlR–GrlAΔ interactions. (a) Pull-down assay to show the binding of GrlAΔ or mutant variants with GrlR. MBP-GrlAΔ proteins were bound to amylose beads, incubated with 6His-GrlR overnight and washed. The eluted proteins were separated by 12.5% SDS–PAGE and the gels stained with Coomassie brilliant blue. The GrlA derivatives employed are indicated above the lanes: MBP-GrlAΔ (R65A K66A), MBP-GrlAΔ (R64A R65A), MBP-GrlAΔ (R53A R54A), WT MBP-GrlAΔ and MBP. (b) Pull-down assay to show the binding of GrlAΔ with GrlR or the GrlR mutants. The GrlR mutants employed are indicated above the lanes: GrlR D17A, GrlR N66A, GrlR S18A, GrlR D35A GrlR E60A and WT GrlR. The input washes and final elution of the representative mutants are shown inSupplementary Fig. S4a. The additional bands seen on the SDS–PAGE (a) were identified as MBP using peptide mass fingerprint analysis (Supplementary Fig. S4b). Western blot analysis of the pull-down assay (a,b) was carried out using anti-MBP and anti-His antibodies (Supplementary Fig. S5a,d). The pull-down results were confirmed in a co-expression, co-purification pETDuet-grlR-grlAΔ system and analysed on a 12.5% native gel (Supplementary Figs S6a,b, S7 and S8). Figure 5: Role of the key residues in the HTH motif region in GrlR–GrlAΔ interactions. ( a ) Pull-down assay to show the binding of GrlAΔ or mutant variants with GrlR. MBP-GrlAΔ proteins were bound to amylose beads, incubated with 6His-GrlR overnight and washed. The eluted proteins were separated by 12.5% SDS–PAGE and the gels stained with Coomassie brilliant blue. The GrlA derivatives employed are indicated above the lanes: MBP-GrlAΔ (R65A K66A), MBP-GrlAΔ (R64A R65A), MBP-GrlAΔ (R53A R54A), WT MBP-GrlAΔ and MBP. ( b ) Pull-down assay to show the binding of GrlAΔ with GrlR or the GrlR mutants. The GrlR mutants employed are indicated above the lanes: GrlR D17A, GrlR N66A, GrlR S18A, GrlR D35A GrlR E60A and WT GrlR. The input washes and final elution of the representative mutants are shown in Supplementary Fig. S4a . The additional bands seen on the SDS–PAGE ( a ) were identified as MBP using peptide mass fingerprint analysis ( Supplementary Fig. S4b ). Western blot analysis of the pull-down assay ( a , b ) was carried out using anti-MBP and anti-His antibodies ( Supplementary Fig. S5a,d ). The pull-down results were confirmed in a co-expression, co-purification pETDuet- grlR-grlA Δ system and analysed on a 12.5% native gel ( Supplementary Figs S6a,b, S7 and S8 ). Full size image ler Promoter region and GrlR compete for HTH motif of GrlA Previous studies demonstrated that GrlA binds to DNA via its HTH motif [10] , and the crystal structure of the GrlR–GrlAΔ complex revealed that GrlR interacts with the HTH motif region of GrlAΔ ( Fig. 3a,b and Supplementary Fig. S2a,b ). On the basis of these observations, we proposed that promoter DNA and GrlR would compete for the HTH motif region of GrlA. To test this prediction, we adopted a structure-guided alanine substitution analysis created in the HTH motif region of full-length MBP-GrlA at the following positions: R53, R54, R64, R65 and K66 of the HTH motif and Y78. Electrophoretic mobility shift assays (EMSAs) were performed to study the interaction of the GrlA mutants with a DNA fragment containing the ler promoter and regulatory regions ( Fig. 6a,b ). Mutants with single alanine substitutions at R53, R54, R65 and K66 exhibited mobility shifts that were less than that observed for the WT GrlA, indicating a reduced affinity for DNA. The MBP-GrlA R64A mutant and a double mutant of MBP-GrlA (R65A K66A) failed to interact with DNA ( Fig. 6b , lanes 4 and 8). Furthermore, the Y78A mutant formed a shifted complex that was comparable to the WT GrlA–DNA complex ( Fig. 6b , lane 7). 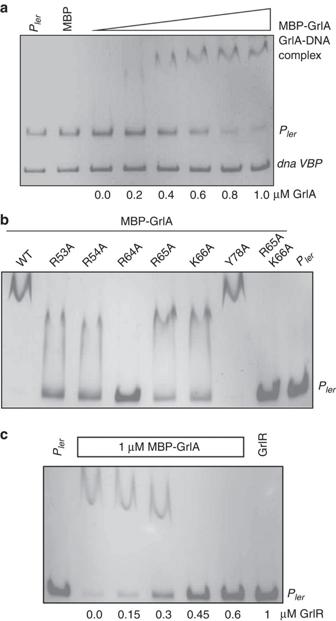Figure 6:Interaction of GrlA with thelerregulatory regionin vitro. (a) EMSA assay for PCR DNA fragments comprising thelerregulatory region (ler−275/+217; numbers indicate the number of base pairs upstream and downstream from the functional ATG start codon, respectively) DNAVBPis a non-specific DNA. (b) EMSA assay with substituted MBP-GrlA proteins. PCR DNA fragments comprising the regulatory region (ler−275/+217) were mixed and incubated with 1.0 μM of purified MBP-GrlA, or with different substituted mutants. Free DNA and protein–DNA complexes were resolved by 5% PAGE and stained with ethidium bromide. The GrlA species used include: WT GrlA, GrlA R53A, GrlA R54A, GrlA R64A, GrlA R65A, GrlA K66A, GrlA Y78A, GrlAR65AK66A andlerpr (ler −275/217). (c) Competitive EMSA assay aimed at testing competition between DNA and 6His-GrlR for binding to MBP-GrlA. PCR DNA fragments comprising the regulatory region (ler−275/+217) were mixed and incubated with 1 μM purified MBP-GrlA for 15 min, then combined with increasing concentrations (0.0, 0.15, 0.3, 0.45 and 0.6 μM) of 6His-GrlR for an additional 15 min. The complexes and free DNA were separated on a 5% native polyacrylamide gel and stained with ethidium bromide (lerpr:ler−275/+217). Figure 6: Interaction of GrlA with the ler regulatory region in vitro. ( a ) EMSA assay for PCR DNA fragments comprising the ler regulatory region ( ler −275/+217; numbers indicate the number of base pairs upstream and downstream from the functional ATG start codon, respectively) DNA VBP is a non-specific DNA. ( b ) EMSA assay with substituted MBP-GrlA proteins. PCR DNA fragments comprising the regulatory region ( ler −275/+217) were mixed and incubated with 1.0 μM of purified MBP-GrlA, or with different substituted mutants. Free DNA and protein–DNA complexes were resolved by 5% PAGE and stained with ethidium bromide. The GrlA species used include: WT GrlA, GrlA R53A, GrlA R54A, GrlA R64A, GrlA R65A, GrlA K66A, GrlA Y78A, GrlAR65AK66A and ler pr (ler −275/217). ( c ) Competitive EMSA assay aimed at testing competition between DNA and 6His-GrlR for binding to MBP-GrlA. PCR DNA fragments comprising the regulatory region ( ler −275/+217) were mixed and incubated with 1 μM purified MBP-GrlA for 15 min, then combined with increasing concentrations (0.0, 0.15, 0.3, 0.45 and 0.6 μM) of 6His-GrlR for an additional 15 min. The complexes and free DNA were separated on a 5% native polyacrylamide gel and stained with ethidium bromide ( ler pr: ler −275/+217). Full size image To determine whether the addition of GrlR could dissociate MBP-GrlA from the ler promoter, a competitive EMSA assay was carried out ( Fig. 6c ). Under the given experimental conditions, when the concentration of GrlR was increased to 0.3 μM, the MBP-GrlA–DNA complex dissociated. No mobility shift of the DNA was detected at higher GrlR concentrations (>0.3 μM). To verify the formation of the GrlR–GrlA complex, a preformed MBP-GrlA–DNA complex bound to amylose beads was titrated against GrlR and washed with DNA-binding buffer. Beads from each of these stages and washes were simultaneously analysed using SDS–polyacrylamide gel electrophoresis (SDS–PAGE) and EMSA assay. The EMSA gel analysis showed no apparent shift in the DNA as compared with DNA alone after the MBP-GrlA–DNA complex was titrated with GrlR ( Supplementary Fig. S9a , lane 6). SDS–PAGE analysis showed bands corresponding to MBP-GrlA and GrlR in the final beads ( Supplementary Fig. S9b , lane 9). These results indicate that DNA bound to MBP-GrlA was replaced by GrlR. Besides, these findings show that GrlR outcompetes with DNA to bind to the GrlA HTH motif. Next, we sought to verify the ability of DNA to pull out GrlA from the GrlR–GrlA complex. A preformed GrlA–GrlR complex was incubated with increasing concentrations of DNA ( P ler ) for about 30 min and then analysed using EMSA assay. There was no apparent shift in the DNA incubated with preformed GrlA–GrlR complex compared with the control DNA fragment ( Supplementary Fig. S10 ). These results clearly show the inability of DNA to displace GrlR from the GrlR–GrlA complex. The GrlR–GrlAΔ complex is functional in vivo We next determined whether the GrlAΔ could form a functional regulatory complex with DNA in vivo . To this end, we employed the EPEC-null strain (Δ grlRA::kn ), which contains a ler-gfp transcriptional fusion (GY2155), and for which the green fluorescent protein (GFP) expression levels report the activity of the ler promoter. This strain was transformed with a plasmid expressing GrlA or GrlAΔ, and the GFP levels were compared by western blot analysis using an antibody directed against GFP. The results show that the activity of the ler promoter in the strain expressing the full-length GrlA and GrlAΔ is almost the same, indicating that GrlAΔ is functional in vivo ( Fig.7a and Supplementary Fig. S11a ). This finding also suggests a negligible role of the last 31 amino acids of GrlA in terms of ler promoter binding. The strain expressing both GrlR and GrlA showed less activity as compared with the strain expressing GrlA alone, illustrating the repressive activity of GrlR. Repression by GrlR in the GrlAΔ-expressing strain was comparable with that expressing both GrlR and full-length GrlA ( Fig.7a and Supplementary Fig. S11a ). 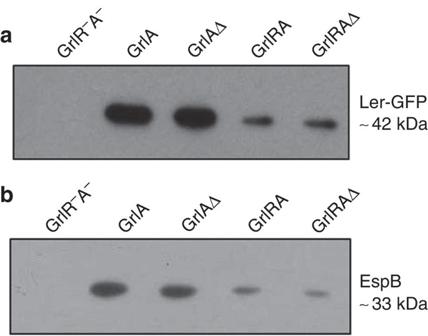Figure 7:In vivofunctionality of GrlR–GrlAΔ asymmetric complex. (a) Immunoblot analysis using anti-GFP antibodies to compare the expression of GFP via thelerpromoter. The used strains include a deletion mutant ofgrlRA(control; indicated as GrlR−A−); this mutant complemented with plasmids expressing GrlA, GrlAΔ, GrlRA and GlRAΔ, as indicted above the lanes. All strains contained a compatible GFP-expressing plasmid via thelerpromoter. (b) Secreted proteins were concentrated from supernatants of bacterial culture grown in DMEM and resolved using 12% SDS–PAGE. These samples were then transferred to a PVDF membrane and analysed using a monoclonal antibody against representative secretory protein EspB. The strains used are as ina, but all lack the GFP-expressing plasmid. Strains are indicated above the lanes as ina. Figure 7: In vivo functionality of GrlR–GrlAΔ asymmetric complex. ( a ) Immunoblot analysis using anti-GFP antibodies to compare the expression of GFP via the ler promoter. The used strains include a deletion mutant of grlRA (control; indicated as GrlR − A − ); this mutant complemented with plasmids expressing GrlA, GrlAΔ, GrlRA and GlRAΔ, as indicted above the lanes. All strains contained a compatible GFP-expressing plasmid via the ler promoter. ( b ) Secreted proteins were concentrated from supernatants of bacterial culture grown in DMEM and resolved using 12% SDS–PAGE. These samples were then transferred to a PVDF membrane and analysed using a monoclonal antibody against representative secretory protein EspB. The strains used are as in a , but all lack the GFP-expressing plasmid. Strains are indicated above the lanes as in a . Full size image An additional readout for the functionality of GrlAΔ is the secretion of EspB, which reflects ler expression and functionality [19] . EspB is a major T3SS effector protein and EspB secretion acts as an indicator for the formation of a functional T3SS [20] . Our measurements of EspB secretion is in agreement with the data obtained with the ler - gfp promoter assay. The secretion assay showed comparable EspB secretion between Δ grlRA::kn -null strains supplemented with a plasmid expressing either GrlAΔ or full-length GrlA ( Fig. 7b and Supplementary Fig. S11b ). Similarly, a comparable amount of EspB was secreted from the mutant expressing GrlRA or GrlRAΔ. Although deletion of the C-terminal region of GrlA resulted in a substantial decrease in the affinity between GrlA and GrlR ( Fig. 4a ), we did not observe significant phenotypic consequences under the experimental conditions used in this study ( Fig. 7a,b and Supplementary Fig. S11a,b ). This suggests that as long as the N-terminal region of GrlA is intact, the protein remains functional. The role of the additional interaction from the C-terminal region of GrlA thus remains to be identified. The key HTH residues are required for GrlA function in vivo EspB secretion was further used to examine the role of the key HTH residues in the regulatory functions of GrlA. To eliminate the negative regulatory effect of GrlR, we transformed the Δ grlRA::kn -null strain with a plasmid expressing GrlAΔ. Bacteria were grown under conditions that favoured positive regulation of the T3SS by GrlA [5] , and the amount of EspB secretion was determined by western blot analysis ( Fig. 8a and Supplementary Fig. S11c ). Secretion of EspB was elevated when the Δ grlRA::kn- null strain was supplemented with GrlAΔ, and GrlA with alanine substitutions at R65 or K66 induced efficient EspB secretion ( Fig. 8a and Supplementary Fig. S11c ). In contrast, the GrlAΔ R64A mutant failed to induce EspB secretion ( Fig. 8a and Supplementary Fig. S11c ) as did the GrlAΔ (R65A K66A) double mutant. Taken together, the results show that substitutions in key residues in the GrlA HTH region, which hamper binding to the ler regulatory region, elicit a profound effect on the ability of the bacteria to assemble a functional T3SS and thus on the bacterial virulence. These effects are presumably related to reduced activity of the ler promoter and consequently reduced expression of some or all of the LEE operons. 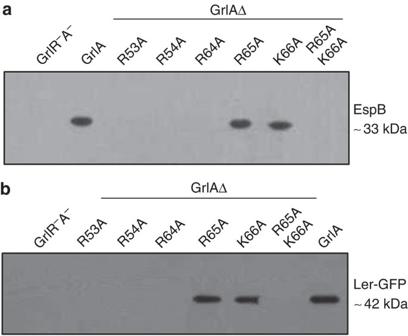Figure 8:In vivoanalysis of the importance of key HTH motif residues in GrlA–DNA binding. (a) Secreted proteins were concentrated from supernatants of bacterial culture grown in DMEM and resolved in 12% SDS–PAGE. The samples were then transferred to a PVDF membrane and analysed using polyclonal antiserum against representative secretory protein EspB. The used strains include a deletion mutant ofgrlRA(control) (indicated as GrlR−A−); this mutant complemented plasmids expressing GrlA or different GrlAΔ substitutions, as indicated above the lanes (b). Immunoblot analysis using anti-GFP antibodies to compare the expression of GFP via thelerpromoter. The used strains are similar to those described ina, with the exception that all contain a compatible GFP expression plasmid via thelerpromoter. Strains are indicated above the lanes. Figure 8: In vivo analysis of the importance of key HTH motif residues in GrlA–DNA binding. ( a ) Secreted proteins were concentrated from supernatants of bacterial culture grown in DMEM and resolved in 12% SDS–PAGE. The samples were then transferred to a PVDF membrane and analysed using polyclonal antiserum against representative secretory protein EspB. The used strains include a deletion mutant of grlRA (control) (indicated as GrlR − A − ); this mutant complemented plasmids expressing GrlA or different GrlAΔ substitutions, as indicated above the lanes ( b ). Immunoblot analysis using anti-GFP antibodies to compare the expression of GFP via the ler promoter. The used strains are similar to those described in a , with the exception that all contain a compatible GFP expression plasmid via the ler promoter. Strains are indicated above the lanes. Full size image To more directly test the role of HTH key residues in the activation of the ler promoter, we employed the ler-gfp promoter assay described above ( Fig. 8b and Supplementary Fig. S11d ). The EPEC-null strain (Δ grlRA::kn ), which contains a ler-gfp transcriptional fusion (GY2155), was transformed with a plasmid expressing various grlA mutants. Substitutions such as R65A and K66A were well tolerated, unlike R54A and R64A, where the activity of the ler promoter was reduced substantially. The results from both the secretion assay and the ler-gfp promoter assays were thus consistent, validating the importance of the key residues in the HTH motif in mediating the function of GrlA as a positive regulator of ler and subsequently as positive regulator of the T3SS biogenesis. GrlR competes with flhDC and ehxCABD operons for GrlA binding We next examined whether the competition between the ler promoter region and GrlR for binding to GrlA was unique to the ler regulatory region or a more general mode of operation of the GrlR–GrlA system. To this end, we examined two additional GrlA targets: the flhDC and ehxCABD promoter regions [11] , [14] , [15] . We performed EMSA assays by incubating MBP-GrlA with a DNA fragment containing the flhDC promoter region. The addition of GrlA shifted the DNA, indicating that MBP-GrlA had bound to the promoter region of the flhDC operon ( Supplementary Fig. S12a ). The HTH mutants that were previously shown to alter GrlA binding to the ler regulatory region showed a similar pattern of binding to the flhDC regulatory region ( Supplementary Fig. S12b ). A competitive EMSA assay also indicated that the addition of GrlR clearly reduced the interaction of GrlA with the flhDC regulatory region, presumably by binding to GrlA and displacing the DNA ( Supplementary Fig. S13 ). With respect to the ehxCABD operon, EMSA assays showed that MBP-GrlA specifically binds to the ehx promoter region. Subsequent EMSA experiments using mutant MBP-GrlA showed various amounts of reduction in the mobility shifts, consistent with those seen for GrlA binding to ler and flhDC promoter regions ( Supplementary Figs S14a–c and S15 ). Cumulatively, our findings suggest that the general mode of operation of the GrlR–GrlA system involves mutually exclusive binding of the GrlA HTH motif with either GrlR or its target DNA. Extensive functional analyses have shown that the GrlR–GrlA is a key regulatory complex involved in the direct or indirect regulation of most virulence genes in AE pathogens, including EPEC, EHEC and C. rodentium [3] , [4] , [6] , [8] . These studies include demonstration of the regulatory role of the GrlR–GrlA system in three independent operons: LEE1 , flhDC and ehxCABD [4] , [11] , [21] . GrlA positively regulates the expression of ler , the first gene in the LEE1 operon, which in turn regulates the expression of various downstream genes involved in T3SS biogenesis [4] . In addition to LEE1 , GrlA is also involved in the positive regulation of ehx operons and the negative regulation of the flhDC operon ( Fig. 1 ). GrlR binds directly to GrlA and functions as an anti-regulator [4] . However, the molecular details of the regulation of the GrlR–GrlA complex have, until now, remained elusive because of the lack of structural details. Here we close this gap, reporting the crystal structure of the GrlR–GrlAΔ complex, along with supportive functional studies. In a previous study, we reported the binding between GrlR and GrlA mediated by the possible interaction of an 46 EDED 49 motif of GrlR with the C-terminal region of GrlA [8] . However, we could not confirm this finding in the present complex structure because of the absence of the C-terminal region (aa107–137) of GrlA in the crystallized construct, wherein the majority of GrlAΔ interactions occurs with one monomer of the dimeric GrlR. Despite this, we were able to verify the binding of full-length GrlA to GrlR using ITC and pull-down experiments ( Fig. 4a , Supplementary Fig. S5c and Supplementary Table. S1 ). The ITC experiments indicated that full-length GrlA binds to GrlR with a ~35-fold higher affinity than GrlAΔ. These results suggest the role of the GrlA C terminus in its interaction with GrlR. Despite this difference in affinity, under the employed experimental conditions, GrlAΔ exhibited an activity comparable to full-length GrlA ( Fig. 7a,b ). Previous studies of the GrlR–GrlA interaction were performed with glutatione S-transferase-tagged proteins [8] , [10] . These studies suggest that the glutathione S-transferase tag might interfere with the interaction, and could be the reason for the complete disruption of GrlA binding with GrlR following alanine substitution in the 46 EDED 49 motif in our previous study [8] . To avoid this potential pitfall, the current experiments were carried out using MBP-tagged GrlA. We and others have independently verified that MBP is not involved in the GrlA–GrlR interaction [10] . Here we show that substitutions in the HTH motif of GrlAΔ interfered with GrlR binding, whereas the full-length GrlA with substitutions in the HTH region was able to bind to GrlR probably through its C-terminal region ( Figs 4b and 5a , Supplementary Fig. S5c ; Supplementary Table S1 ). Jimenez et al. [10] show that GrlAΔ [1] (aa1–100) was able to pull down GrlR, and our observation of two binding sites agrees with this finding. Thus, even though the binding site located to the GrlA C terminus was deleted, these deletion constructs can still pull down GrlR via this alternative binding site located at the HTH region. Our data shows that GrlR interacts with GrlA to prevent its binding to target DNA. The fact that grlR and grlA are co-transcribed raises the question that under what conditions GrlA can escape suppression by GrlR and interact with its target DNA. Given the tight GrlR–GrlA mode of interaction and the observation that two GrlR molecules are to needed suppress one GrlA molecule, it can be assumed that GrlA will function as a regulator only when its steady-state level reaches more than half of that for GrlR. The relative steady-state level of the two proteins is controlled by their relative translation rates and stability. Although virtually nothing is known about the first, it is expected that the translation rate would be equal in generating both GrlR bound, as well as free, GrlA. The differential stability and specific GrlR degradation by ClpXP has been previously reported [6] . An additional point of view on this system is that GrlR in complex with GrlA stabilizes GrlA and maintains it in an inactive state that can become functional and rapidly released following an appropriate signal and ClpXP-mediated GrlR degradation. In conclusion, the present study revealed the molecular structure and mechanism of the GrlR–GrlA complex. GrlR and the promoter regions of ler , flhDC and ehxCABD compete for the HTH motif region of GrlA. GrlR outcompetes with these promoter DNA sequences for GrlA. Regulation of multiple virulence operons by a central heterotrimeric GrlR–GrlA complex would help the pathogen to precisely control the expression of various genes involved in its pathogenesis. By differentially regulating the ler and ehx operons positively and the flhDC operon negatively, GrlR and GrlA coordinate and optimize gene expression by the pathogen during the infection process. Plasmid and strain construction Bacterial strains and plasmids used in this study are listed in Supplementary Table S2 . Intact grlR and grlA genes were PCR-amplified from EHEC EDL933 (ref. 22 ) chromosomal DNA and cloned into MCS1 (with a 6His tag) and MCS2 of the pETDuet-1 (Novagen, Madison, WI, USA) vector, respectively. Plasmid pET32- grlR was constructed by amplifying the grlR gene from EHEC EDL933 chromosomal DNA and cloning into pET32 vector. Plasmid pGEX- grlA and pMBP- grlA were constructed by amplifying the grlA DNA fragments from EHEC EDL933 chromosomal DNA and cloning into pGEX-4T1 (GE Healthcare, Buckinghamshire, UK) and pMAL-c2X (New England Biolabs, Ipswich, MA, USA), respectively. The EPEC grlRA- null mutant (Δ grlRA ::kn) was constructed by replacing the grlRA gene from an EPEC strain with a kanamycin cassette by the one-step method using the λ -recombinase system [23] . Site-specific mutations in grlA were introduced by overlapping PCR [24] , which uses complementary oligodeoxyribonucleotide (oligo) primers and the PCR to generate two DNA fragments having overlapping ends. These fragments are annealed, allowing the 3′-overlap of each strand to serve as a primer for the 3′-extension of the complementary strand. The resulting fusion product is amplified further by PCR. Specific mutations in the nucleotide sequence were introduced by incorporating nucleotide changes into the overlapping oligo primers. Each construct was verified by DNA sequencing. To construct pGY1, a DNA fragment containing P LEE1 and ler (starting from position −159 compared with the transcriptional start site) was amplified using specific primers; this amplified fragment was digested by Xba I and Bam HI and cloned into pIR1 digested by the same enzymes [20] , [25] . The null strain (Δ grlRA ::kn) transformed with pGY1 was named GY2155. GrlR–GrlAΔ complex structure determination pETDuet1- grlR-grlA Δ plasmid was transformed into E. coli BL21 cells and grown in defined M9 medium [26] supplemented with 25 mg l −1 L-SeMet at 37 °C until the optical density reached 0.6 at 600 nm. A 1-litre culture was induced with 100 μM isopropyl β- D -1-thiogalactopyranoside and grown overnight at 20 °C. Cells were then collected by centrifugation and resuspended in 40 ml of lysis buffer (50 mM Tris-HCl (pH 7.0), 0.2 M NaCl, 1% (w/v) Triton X-100, 5% (w/v) glycerol, 10 mM β-mercaptoethanol) with complete protease inhibitors (Roche Applied Science, Mannheim, Germany). The GrlA–GrlRΔ complex was purified in two steps using Ni-NTA (Qiagen, Valencia, CA, USA), followed by gel filtration (Superdex75, GE Healthcare). The 6His tag remained intact on GrlR. Drops containing 1 μl of protein solution (7 mg ml −1 ) and 1 μl of reservoir solution were equilibrated by hanging-drop vapour diffusion at 25 °C. The best crystals were grown from 12% PEG 3350, 0.1 M sodium malonate pH 5 and 0.4 M non-detergent sulphobetaines 201, with the protein in 30 mM Tris-HCl (pH 7.0), 200 mM NaCl and 5% (w/v) glycerol. One complex consisted of two GrlR and one GrlAΔ (2:1) molecule in the asymmetric unit, which accounts for a Matthews coefficient of 2.40 Å 3 Da −1 (ref. 27 ), corresponding to a solvent content of 49%. Crystals were cryoprotected in the reservoir solution supplemented with 25% glycerol and flash cooled at 100 K. The structure was determined using SeMet-labelled protein crystals by single-wavelength anomalous dispersion [28] . X-ray diffraction data were collected at beamline 13B1, National Synchrotron Radiation Research Centre (Taiwan), using a Quantum-315r charge-coupled device area detector (ADSC) and processed with HKL2000 (ref. 29 ). All of the expected eight Se sites of an asymmetric unit were located using the programme Phenix-Autosol. The phases were further improved by density modification using RESOLVE [30] , which gave a final overall figure of merit of 0.70. Over 50% of the backbone atoms of the model were built by RESOLVE. The remaining residues were manually built using COOT [31] and refined with phenix-refine [32] . Refinement was continued until the R -value converged to 0.18 ( R free =0.23) for reflections I> σ (I) to 2.7 Å resolution ( Table 1 ). The model had good stereochemistry, with 99.3% residues falling within the allowed regions of the Ramachandran plot. Subsequently, the importance of the key residues in the HTH motif region was validated by structure-based in vitro studies, such as ITC and pull-down assay (see Supplementary Methods ). Analytical ultracentrifugation The stoichiometric ratio of WT GrlR–GrlA complex was investigated by monitoring their sedimentation properties in sedimentation velocity experiments. Samples (400 μl) were used at A 280 nm of 1.0 in 30 mM Tris-HCl (pH 7.0), 200 mM NaCl and 5% glycerol. Sedimentation velocity profiles were collected by monitoring the absorbance at 280 nm. The samples were sedimented at 40,000 r.p.m. at 20 °C in a Beckman Optima XL-I centrifuge (Beckman Coulter Inc., Brea, CA, USA) fitted with a four-hole AN-60 rotor and double-sector aluminium centre pieces, and equipped with absorbance optics. A total of 200 scans were collected and analysed using the Sedfit programme [33] . Circular dichroism spectrometry Far ultraviolet spectra (260–190 nm) of MBP-GrlA/MBP-GrlAΔ and its substituents were measured using a Jasco J-810 spectropolarimeter (Jasco Europe, Milan, Italy) in phosphate buffer (pH 7.5) at room temperature using a 0.1-cm path length and stoppered cuvettes. Six scans were recorded, averaged and the baseline subtracted. Isothermal titration calorimetry MBP-GrlA, MBP-GrlAΔ (with or without substitutions in the HTH motif region) and GrlR were all purified in gel filtration buffer containing 30 mM Tris-HCl (pH 7.0), 200 mM NaCl and 5% glycerol. ITC experiments were carried out using a VP-ITC calorimeter (Microcal, LLC, Northampton, MA, USA) at 25 °C using 0.01 mM protein (MBP-GrlA/MBP-GrlAΔ) in the sample cell and 0.15–0.22 mM GrlR in the injector. All samples were thoroughly degassed and then centrifuged to remove precipitates. Excluding the first 2-μl injection, 10-μl injections were sequentially made in each experiment. Consecutive injections were separated by 5 min to allow the peak to return to baseline levels. ITC data were analysed with a model considering a single class of binding sites implemented in Origin 7.0 (Origin Lab Corp., Northampton, MA, USA) software. Electrophoretic mobility shift assays EMSA assays were performed by mixing ~100 ng of DNA (promoter region of ler (−275/+217; numbers indicate the number of base pairs upstream and downstream from the functional ATG start codon, respectively), flhDC (−455/+223) or ehxCABD (−261/+22) with increasing concentrations of purified WT or mutant MBP-GrlA proteins in binding buffer containing 10 mM Tris-HCl (pH 8), 50 mM KCl, 1 mM dithiothreitol, 0.5 mM EDTA, 10 μg ml −1 BSA and 5% glycerol. The primers used to amplify the promoter regions are shown in Supplementary Table S3 . Reaction mixtures were incubated for 30 min at room temperature and then separated by electrophoresis on 5% polyacrylamide gels in 0.5 × Tris-borate–EDTA buffer. DNA bands were stained with ethidium bromide and visualized with a Syngene transilluminator (Syngene, Frederick, MD, USA). For competitive EMSA assays, DNA was incubated with 1 μM MBP-GrlA for 30 min, followed by the addition of increasing concentrations of His-GrlR for an additional 30 min at room temperature. The complexes were visualized as described above. The formation of GrlR–GrlA complex in the competitive EMSA assay was verified by setting up a 300-μl amylose-resin-bound MBP-GrlA–DNA-binding reaction for 30 min. A 30-μl sample was run as input on EMSA assay and SDS–PAGE, and the rest was washed several times with excess DNA-binding buffer before titrating with GrlR. A 30-μl sample was run after titrating with GrlR followed by washes. The final beads and all other washes along with the initial samples were analysed on both EMSA and SDS–PAGE gels. All the EMSA studies were repeated three times and the results were consistent. Extracellular protein extraction and detection Overnight cultures of EPEC strains were grown in DMEM medium (Invitrogen, Carlsbad, CA, USA) and supplemented with 30 μg ml −1 of kanamycin, 40 μg ml −1 streptomycin and 34 μg ml −1 chloramphenicol until the optical density at 600 nm reached 0.8. The cultures were diluted 1:50 into fresh DMEM medium and incubated for 9 h at 37 °C in a shaking water bath at 200 r.p.m. Bacterial cells were centrifuged at 5,500 g for 10 min at 4 °C and the supernatants were passed through a 0.22-μm filter (Millex, Millipore). The extracellular protein fraction was isolated by trichloroacetic acid precipitation and the protein pellet was washed thrice with −20 °C acetone and then air dried [34] . Extracellular protein pellets were solubilized in Ready Prep reagent 3 (5 M urea, 2 M thiourea, 2% (w/v) CHAPS, 2% (w/v) SB 3–10, 40 mM Tris and 0.2% (w/v) Bio-Lyte 3/10 ampholyte (Bio-Rad, Hercules, CA, USA)), and stored at −80 °C, as described [34] . Proteins were transferred to a polyvinylidene difluoride (PVDF) membrane. EspB was detected by the addition of diluted anti-EspB (1:2,000) polyclonal antiserum, followed by a 1:5,000 dilution of mouse anti-rabbit IgG horseradish peroxidase (1:5,000; Santa Cruz Biotechnology, Santa Cruz, CA, USA). The PVDF membrane was examined using the SuperSignal WestPico Chemiluminescent substrate (Pierce Biotechnology; Rockford, IL, USA) under the conditions recommended by the manufacturer. ler-gfp Promoter assay The plasmid pGY1 contains a transcriptional fusion of the gfp to the ler gene and its regulatory region [20] . The plasmid was transformed into the EPEC grlRA::kn mutant strain EM3715 to create strain GY2155. EPEC strain GY2155 was then transformed with a compatible, pACYC184-based plasmid, expressing GrlA or GrlAΔ and various grlA mutants. The constructed strains were grown in DMEM overnight as described above. Cells were then collected by centrifugation at 5,500 g for 10 min at 4 °C and resuspended in lysis buffer (1 × PBS) with complete protease inhibitors (Roche Applied Science). The cells were lysed and centrifuged down at 30,000 g for 30 min. Protein concentrations in the supernatant were adjusted and separated on an SDS–PAGE, transferred to a PVDF membrane and subjected to western blotting. GFP was detected by the addition of diluted anti-GFP (1:2,000) rabbit monoclonal antibody (Invitrogen), followed by a 1:5,000 dilution of mouse anti-rabbit IgG horseradish peroxidase (Santa Cruz Biotechnology). The PVDF membrane was examined using the SuperSignal WestPico Chemiluminescent substrate under the conditions recommended by the manufacturer. Accession code: Coordinates of GrlR:GrlAΔ complex have been deposited in the Protein Data Bank under accession code 4KT5 . How to cite this article: Padavannil, A. et al. Structure of GrlR–GrlA complex that prevents GrlA activation of virulence genes. Nat. Commun. 4:2546 doi: 10.1038/ncomms3546 (2013).